Dry-air-stable lithium silicide–lithium oxide core–shell nanoparticles as high-capacity prelithiation reagents Rapid progress has been made in realizing battery electrode materials with high capacity and long-term cyclability in the past decade. However, low first-cycle Coulombic efficiency as a result of the formation of a solid electrolyte interphase and Li trapping at the anodes, remains unresolved. Here we report Li x Si–Li 2 O core–shell nanoparticles as an excellent prelithiation reagent with high specific capacity to compensate the first-cycle capacity loss. These nanoparticles are produced via a one-step thermal alloying process. Li x Si–Li 2 O core–shell nanoparticles are processible in a slurry and exhibit high capacity under dry-air conditions with the protection of a Li 2 O passivation shell, indicating that these nanoparticles are potentially compatible with industrial battery fabrication processes. Both Si and graphite anodes are successfully prelithiated with these nanoparticles to achieve high first-cycle Coulombic efficiencies of 94% to >100%. The Li x Si–Li 2 O core–shell nanoparticles enable the practical implementation of high-performance electrode materials in lithium-ion batteries. Rechargeable lithium-ion batteries are widely used for consumer electronics and exhibit great potential for electrical vehicle and grid-scale energy storage [1] , [2] , [3] , [4] . The first charging process, in which lithium ions and electrons move from cathode to anode, is critical for lithium-ion battery operation. When the potential of the anode is below ~1 V versus Li metal, the organic electrolyte is reduced on the anode surface to form a layer of solid electrolyte interphase (SEI) that consists of a complex composition of inorganic and organic lithium compounds [5] , [6] , [7] , [8] . In addition, some lithium may be trapped in the electrode upon lithiation [9] . As a result, the first charging process irreversibly consumes a fraction of the lithium ions, giving rise to a net loss of storage capacity. Such first-cycle irreversible capacity loss is usually compensated by additional loading of cathode materials in current lithium-ion batteries. However, lithium metal-oxide cathodes have much lower specific capacity (mostly less than ~200 mAh g −1 ) than anodes [3] , [10] . Excessive loading of cathode material causes appreciable reduction of battery specific energy and energy density. It is therefore attractive to develop an alternative method that suppresses this loss and consequently increases the first-cycle Coulombic efficiency. Addressing first-cycle capacity loss is an important step forward in the success of commercial graphite anodes. With graphite anodes, 5–20% of the lithium from the cathode is consumed to form the SEI, corresponding to an appreciable amount of inactivated cathode material. In the past two decades, the first-cycle Coulombic efficiency of graphite anodes has increased from <80% to 90–95% through optimization of material quality, electrolyte and additives [11] , [12] , [13] , [14] . Further improvement is likely to result from pre-compensation or prelithiation of the electrodes [15] . Besides graphite anodes, prelithiation presents exciting opportunities for next-generation high-capacity anode materials such as Si, Ge and Sn, which have a large first-cycle capacity loss [16] , [17] . For example, Si is a particularly attractive anode material, owing to its high specific capacity of ~4,200 mAh g −1 , excellent material abundance and well-developed industrial infrastructure for manufacturing [16] , [18] . In the past several years, there has been exciting progress in addressing the issues associated with large volume change (>300%) during lithium insertion and extraction by designing nanostructured Si including nanowires and core–shell nanowires [19] , [20] , [21] , [22] , hollow particles and tubes [23] , [24] , [25] , porous materials [26] , [27] , Si/C nanocomposites [28] , [29] , [30] and by using novel binders [31] , [32] , [33] , [34] . One of the remaining issues for Si anodes is the large capacity loss in the first cycle. The first-cycle Coulombic efficiency is typically very low, in the range of 50–80% [31] , [35] , [36] , [37] , in spite of a few reports with higher values of ~85% [38] , [39] . The first-cycle Coulombic efficiency can be improved by prelithiation. Anode prelithiation has been previously achieved by inducing electrical shorting between anode materials and lithium metal foil [40] , [41] . It requires a temporary battery to be fabricated, a process that is difficult to scale up. In addition, prelithiation of a thick electrode with Li foil is time consuming, as it requires the diffusion of Li ions across the entire anode. Another approach is to use stabilized lithium metal powder (SLMP), which is effective to pre-compensate the first-cycle irreversible capacity loss of different anode materials, such as graphite and silicon-carbon nanotube (Si–CNT) composite [15] , [42] , [43] , [44] . It is thus far the only prelithiation reagent in the powder form that can potentially be adopted during battery manufacturing, although practical challenges still exist to be addressed [45] . It is therefore highly desirable to develop alternative microparticles or nanoparticles (NPs) for prelithiation. Herein, we demonstrate that chemically synthesized core–shell NPs of Li x Si–Li 2 O ( Fig. 1 ) as an excellent prelithiation reagent, which can be mixed with various anode materials during slurry processing. Li x Si NPs exhibit multiple attractive properties for prelithiation: (1) fully lithiated Li x Si alloy has a sufficiently low potential of around 10 mV versus Li/Li + to prelithiate all types of anodes including graphite, Si, Ge and Sn [16] , [18] , [46] ; (2) Li x Si has very high specific capacity (4,200 mAh g −1 of Si, 2,000 mAh g −1 of Li 4.4 Si) for pre-storing lithium, so only a small percentage of material is needed for prelithiation; (3) nanoscale Li x Si–Li 2 O particles (100~200 nm) are helpful for distributing pre-stored Li uniformly across the anodes. Furthermore, using nanoscale Li x Si–Li 2 O particles as prelihitation reagent is less likely to disturb the whole structure of the electrode [47] ; (4) nanoscale Li x Si particles provide a localized lithium source to realize fast prelithiation of anode materials, compared with the process of inducing electrical shorting between anode materials and lithium metal foil; (5) potentially, Li x Si can be benefit from the mature manufacturing infrastructure of the Si industry for scale-up and low-cost manufacturing. 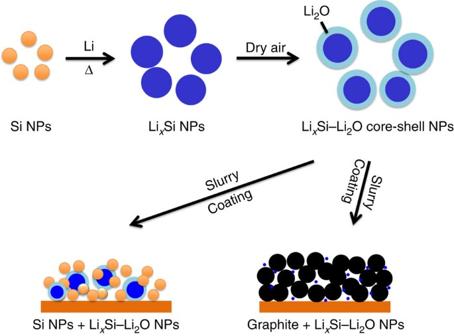Figure 1: Schematic diagrams showing Si NPs react with melted Li to form LixSi NPs. A dense passivation layer is formed on the LixSi NPs after exposure to trace amounts of oxygen, preventing the LixSi alloy from further oxidation in dry air. As-synthesized LixSi–Li2O core–shell NPs, compatible with the existing battery-manufacturing environment, can be mixed with various anode materials during slurry processing and serve as an excellent prelithiation reagent. Figure 1: Schematic diagrams showing Si NPs react with melted Li to form Li x Si NPs. A dense passivation layer is formed on the Li x Si NPs after exposure to trace amounts of oxygen, preventing the Li x Si alloy from further oxidation in dry air. As-synthesized Li x Si–Li 2 O core–shell NPs, compatible with the existing battery-manufacturing environment, can be mixed with various anode materials during slurry processing and serve as an excellent prelithiation reagent. Full size image Another challenge associated with anode prelithiation is the high chemical reactivity of prelithiation reagents, which make them difficult to survive multiple processing steps (exposure to air and solvents, slurry mixing, coating and baking) during battery electrode fabrication. A protective coating is therefore needed. However, this coating needs to be activated later to ensure quick lithium-ion diffusion for prelithiation. Li x Si is a very reactive prelithiation reagent. In this paper, we also studied how to protect and de-protect it using a Li x Si–Li 2 O core–shell nanostructure. The following findings in this paper are important to enable successful prelithiation: (1) The core–shell NPs rapidly react with solvents containing active protons such as water and alcohol. The slow reaction with oxygen, however, allows the formation of a dense Li 2 O shell that protects the Li x Si core in dry-air environments over the long term. This is exciting since these NPs are compatible with the low-humidity environment of a dry room, commonly used in existing battery manufacturing; (2) for solvents without active protons, we found that Li x Si can survive in low-polarity solvents such as ether and toluene during slurry processing. Highly polar solvents such as N -methyl-2-pyrrolidinone and organic carbonate can weaken the protection of the Li 2 O shell and react with the Li x Si core, making them poor candidates for solvents in slurry processing. At the end of the battery assembly process, carbonate electrolyte is injected, directly resulting in the activation of the facile lithium diffusion into anode materials. To the best of our knowledge, this is the first report on prelithiation of anode materials with stabilized Li x Si NPs. Synthesis and characterizations of Li x Si–Li 2 O NPs Li x Si NPs were synthesized by mechanical stirring of a stoichiometric mixture (1:4.4) of Si NPs (~50 nm in diameter) and Li metal foil at 200 °C for 6 h in a glove box (Ar-atmosphere, H 2 O level <0.1 p.p.m. and O 2 level <3 p.p.m.). In the process, the colour of the powder changes from brown to black, indicating the formation of the Li x Si alloy. Owing to trace oxygen in the glove box, a dense Li 2 O passivation layer will form outside the Li x Si NPs, resulting in the formation of Li x Si–Li 2 O core–shell NPs and preventing Li x Si from further oxidizing. The Li 2 O passivation layer was evidenced by extensive characterization. Transmission electron microscopy (TEM) images were taken immediately after exposure of the samples to the electron beam to minimize the impact of the electron beam on the NPs. The TEM image ( Fig. 2a ) and scanning electron microscopy (SEM) image ( Supplementary Fig. 1a ) show that the size of the Li x Si NPs range from 100 to 200 nm, which is larger than the Si NPs (50 nm) due to volume expansion and some aggregation of particles during the alloying process. The magnified TEM image ( Fig. 2b ) shows a thin passivation layer (~10 nm thick) on the surface of the Li x Si NPs. 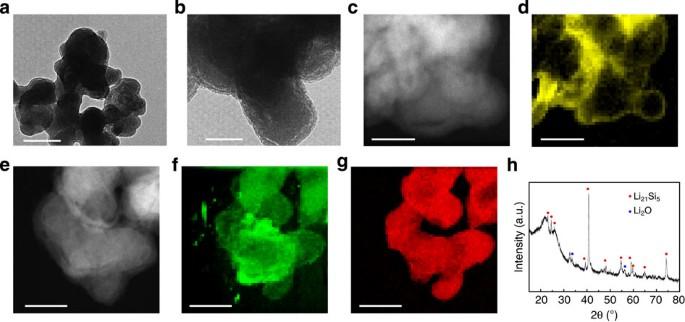Figure 2: Characterization of LixSi–Li2O core–shell NPs. (a) TEM image of LixSi–Li2O NPs. Scale bar, 200 nm. (b) Magnified TEM image reveals the core–shell nanostructure. (c) STEM image of LixSi–Li2O NPs, and (d) the corresponding EELS map of O distribution. Scale bar, 100 nm (b–d). (e) STEM image of LixSi–Li2O NPs. Corresponding EELS maps of (f) Li distribution and (g) Si distribution. Scale bar, 200 nm (e–g). (h) XRD pattern reveals the core–shell nanoparticles consisting of crystalline Li21Si5and Li2O. Figure 2: Characterization of Li x Si–Li 2 O core–shell NPs. ( a ) TEM image of Li x Si–Li 2 O NPs. Scale bar, 200 nm. ( b ) Magnified TEM image reveals the core–shell nanostructure. ( c ) STEM image of Li x Si–Li 2 O NPs, and ( d ) the corresponding EELS map of O distribution. Scale bar, 100 nm ( b – d ). ( e ) STEM image of Li x Si–Li 2 O NPs. Corresponding EELS maps of ( f ) Li distribution and ( g ) Si distribution. Scale bar, 200 nm ( e – g ). ( h ) XRD pattern reveals the core–shell nanoparticles consisting of crystalline Li 21 Si 5 and Li 2 O. Full size image Compositional analysis of the Li x Si NPs was acquired by electron energy loss spectroscopy (EELS) in the TEM. EELS is ideal for Li mapping, since the shallow Li K-edge has a high-ionization cross-section, which is about 10–100 times greater than that of other light elements such as oxygen [48] . Oxygen mapping is therefore performed with longer exposure time per step. Compared with the scanning transmission electron microscopy (STEM) image in Fig. 2c , the corresponding EELS oxygen map ( Fig. 2d ) reveals that oxygen is concentrated in the passivation layer of the core–shell NPs. To avoid possible beam damage through consecutive scans, a different region is selected for Li and Si mapping. STEM image ( Fig. 2e ) and corresponding EELS elemental mapping reveal the spatial distribution of Li ( Fig. 2f ) and Si ( Fig. 2g ), respectively. The specific electron energy loss spectra of Li, Si and O are shown in Supplementary Fig. 2 . According to the elemental maps, Li is distributed throughout the entire nanoparticle, whereas Si is distributed in the internal part of the nanoparticle. Both images and elemental maps suggest that the NPs form a core–shell structure, consisting of a core of Li x Si and a shell of Li 2 O. Furthermore, X-ray diffraction (XRD) of the product ( Fig. 2h ) reveals the crystalline nature of the core–shell NPs formed by Li 21 Si 5 (PDF# 00-018-747) and Li 2 O (PDF# 04-001-8930). The broad background comes from the Kapton tape used to protect the samples from moisture in the air. Li 21 Si 5 , a variation of the Li 22 Si 5 phase with ordered vacancies, is the most thermally stable phase among the crystalline lithium silicides [46] , [49] . Electrochemical performance To study the electrochemical properties of the Li x Si–Li 2 O NPs, half cells were fabricated with Li metal as a counter electrode. LiPF 6 (1.0 M) in a mixture of 1:1 w/w ethylene carbonate/diethyl carbonate, 10 vol% fluoroethylene carbonate and 1 vol% vinylene carbonate was used as the electrolyte. To find a proper solvent for the slurry process, Li x Si–Li 2 O NPs were mixed with carbon black (Super P) and polyvinylidene fluoride (PVDF) (65:20:15 by weight) in different solvents to form a slurry, which was then drop cast on copper foil and dried under vacuum. The entire battery electrode preparation process from the slurry formation to drop casting and drying were performed in a dry-air glove box (dew point=−50 °C). The capacities of the resulting electrodes were studied by delithiating the samples to 1 V directly. 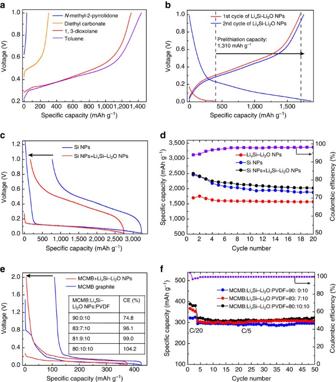Figure 3: Electrochemical characteristics. (a) First-cycle delithiation capacity of LixSi–Li2O NPs, using different solvents to form the slurry. (b) Galvanostatic discharge/charge profiles of LixSi–Li2O NPs in first and second cycles. (c) First-cycle voltage profiles of Si NPs/LixSi–Li2O and Si NPs show that the incorporation of LixSi–Li2O additive compensates the first-cycle capacity loss of Si NPs. (d) Cycling performance of LixSi–Li2O NPs, Si NPs/LixSi–Li2O and the control Si NPs at C/20 (1C=4.2 A g−1Si, the capacity is based on the total mass of Si in the electrodes). The purple line is the Coulombic efficiency of Si NPs/LixSi–Li2O composite. (e) First-cycle voltage profiles of MCMB/LixSi–Li2O (81:9 by weight) show LixSi–Li2O NPs improve the first-cycle Coulombic efficiency of MCMB. The table shows that the first-cycle Coulombic efficiency is tuned by the amount of LixSi–Li2O additives. (f) Cycling performance of MCMB/LixSi–Li2O composites with different weight ratios at C/20 for first three cycles and C/5 for the following cycles (1C=0.372 A g−1C, the capacity is based on the mass of the total active materials, including MCMB and Si in LixSi–Li2O NPs). The purple line is the Coulombic efficiency of MCMB/LixSi–Li2O composite (80:10 by weight). Figure 3a shows that there is almost no Li capacity extracted from the Li x Si–Li 2 O NPs processed with N -methyl-2-pyrrolidinone solvent. With diethyl carbonate solvent, the Li x Si–Li 2 O NPs show a small Li extraction capacity of ~300 mAh g −1 , indicating that most of the stored Li is not active. Excitingly, Li x Si–Li 2 O NPs are compatible with 1,3-dioxolane (DOL) and toluene ( Fig. 3a ), showing high extraction capacities of 1,200–1,400 mAh g −1 , which is sufficient to qualify it as a prelithiation reagent. It appears the highly polar functional groups can be attacked by free electrons in Li x Si acting as a nucleophile. The detailed reaction mechanism is shown in Supplementary Fig. 3 . Notice that PVDF binder does not dissolve in toluene to form a uniform slurry, so DOL is selected in the following experiments. Figure 3: Electrochemical characteristics. ( a ) First-cycle delithiation capacity of Li x Si–Li 2 O NPs, using different solvents to form the slurry. ( b ) Galvanostatic discharge/charge profiles of Li x Si–Li 2 O NPs in first and second cycles. ( c ) First-cycle voltage profiles of Si NPs/Li x Si–Li 2 O and Si NPs show that the incorporation of Li x Si–Li 2 O additive compensates the first-cycle capacity loss of Si NPs. ( d ) Cycling performance of Li x Si–Li 2 O NPs, Si NPs/Li x Si–Li 2 O and the control Si NPs at C/20 (1C=4.2 A g −1 Si, the capacity is based on the total mass of Si in the electrodes). The purple line is the Coulombic efficiency of Si NPs/Li x Si–Li 2 O composite. ( e ) First-cycle voltage profiles of MCMB/Li x Si–Li 2 O (81:9 by weight) show Li x Si–Li 2 O NPs improve the first-cycle Coulombic efficiency of MCMB. The table shows that the first-cycle Coulombic efficiency is tuned by the amount of Li x Si–Li 2 O additives. ( f ) Cycling performance of MCMB/Li x Si–Li 2 O composites with different weight ratios at C/20 for first three cycles and C/5 for the following cycles (1C=0.372 A g −1 C, the capacity is based on the mass of the total active materials, including MCMB and Si in Li x Si–Li 2 O NPs). The purple line is the Coulombic efficiency of MCMB/Li x Si–Li 2 O composite (80:10 by weight). Full size image To evaluate the electrochemical behaviour of the Li x Si–Li 2 O NPs, normal deep galvanostatic lithiation/delithiation was used. Figure 3b shows the voltage profiles of the first and second cycles. Li x Si–Li 2 O NPs were first lithiated to 0.01 V, and then delithiated to 1 V at a rate of C/20 (the specific capacity is calculated based on the mass of Si in the electrode. 1C=4.2 A g −1 Si). The open-circuit voltage (OCV) of Li x Si–Li 2 O NPs was <0.2 V, which is significantly lower than that of crystalline Si NPs. The capacity preloaded into Si NPs is 1,310 mAh g −1 , determined by subtracting the first lithiation capacity from the delithiation capacity. After the first cycle, the voltage profile is similar to normal Si anodes, but the second-cycle Coulombic efficiency of the Li x Si–Li 2 O NPs is 96%, still higher than that of Si NPs (93%) ( Supplementary Fig. 5a ). During the slurry process, we believe that DOL will decompose on the surface of the Li x Si–Li 2 O core–shell NPs to form a thin coating due to the strong reducing power of Li x Si ( Supplementary Fig. 1b ). The reaction only consumes part of the Li stored in the Li x Si–Li 2 O NPs, and a significant amount of electrochemically active Li is left to be used as the prelithiation reagent. Figure 3c demonstrates that Li x Si–Li 2 O NPs can be used as a prelithiation reagent to improve the first-cycle Coulombic efficiency of normal Si NP anodes. The anodes were made by forming a slurry of Si NPs, Li x Si–Li 2 O NPs, carbon black and PVDF binder with a mass ratio of 50:15:20:15. The dimensions of the Li x Si–Li 2 O NPs are the same as that of Si NPs, so the Li x Si–Li 2 O NPs were more uniformly distributed in the electrode compared with large-size prelithiation reagent. After a coin cell was fabricated, 6 h was needed for the anode to reach equilibrium. The first-cycle voltage profile reveals an OCV of 0.27 V, much lower than that of the control cell, which indicates partial prelithiation of the Si NPs. The capacity of the Li x Si–Li 2 O NPs compensates the irreversible capacity loss of the Si NPs in the first cycle. Therefore, the first-cycle Coulombic efficiency increased from 76 to 94%. In addition, the lithiation capacity due to SEI formation decreases, due to the pre-formation of SEI during the prelithiation process. The electrochemical cycling performance was evaluated using deep lithiation/delithiation cycling from 1 to 0.01 V. The Li x Si–Li 2 O NPs exhibited improved cycling performance over Si NPs at C/20 as displayed in Fig. 3d . Using Li x Si–Li 2 O NPs as anode material, enough void space formed during the delithiation will be pre-built into the electrode structure to accommodate the volume expansion during the next lithiation process. Accordingly, the introduction of Li x Si–Li 2 O NPs into Si NP anodes did not affect the cycling performance of Si NPs (the specific capacity was based on the total mass of Si in the electrode. 1C=4.2 A g −1 Si). The cyclic voltammetry (CV) measurement of Si/Li x Si–Li 2 O NPs ( Supplementary Fig. 4b ) also demonstrates the performance of Si anode is negligibly affected by the addition of prelithiation reagents. Li x Si–Li 2 O NPs can also be used to compensate the irreversible capacity loss of existing graphite anodes as shown in the first-cycle voltage profiles ( Fig. 3e ). Graphite anodes consisting of mesocarbon microbeads (MCMB) graphite and a PVDF binder (90:10 by weight) were measured in a voltage window from 0.005 to 2 V as a control. In Fig. 3e , the blue voltage profile reveals a sloping region between 0.7 and 0.2 V, corresponding to SEI formation during first-cycle lithiation. As a result, the apparent first lithiation capacity of MCMB graphite is higher than the theoretical capacity of graphite (372 mAh g −1 ), whereas the first-cycle Coulombic efficiency is just 75%. Prelithiation of the MCMB graphite by Li x Si–Li 2 O NPs (mass ratio 81:9, red line) yields a first-cycle Coulombic efficiency of 99%. The electrochemical potential of the electrode is close to 0.3 V, indicating partial prelithiation of MCMB graphite. The incorporation of Li x Si–Li 2 O NPs decreases the typical lithiation capacity, due to the pre-formation of SEI during the prelithiation process. CV of MCMB/Li x Si–Li 2 O composites (blue) and MCMB graphite (red) shows consistent results ( Supplementary Fig. 4c ). As shown in the table in Fig. 3e , the first-cycle Coulombic efficiency of MCMB anodes can be adjusted by tuning the amount of Li x Si–Li 2 O additive. The first-cycle Coulombic efficiency ranges from 96 to 104% by varying the mass ratio of MCMB to Li x Si–Li 2 O NPs from 83:7 to 80:10. The MCMB/Li x Si–Li 2 O composites (mass ratio of 83:7 and 80:10) exhibited stable cycling performance at C/20 for the first three cycles and C/5 for the following cycles (1C=372 mA g −1 C) as displayed in Fig. 3f . The specific capacity was based on the mass of MCMB graphite and Si in the Li x Si–Li 2 O additives. The capacities of MCMB/Li x Si–Li 2 O composites are slightly higher than that of the control graphite cell, contributed by the capacity stored in the Li x Si–Li 2 O NPs. The incorporation of Li x Si–Li 2 O NPs into the MCMB graphite electrode does not damage the structure of the electrode during cycling. As a result, the cycling performance of MCMB graphite is not affected. Furthermore, Li x Si–Li 2 O additives also improve the second-cycle Coulombic efficiency of MCMB, and Coulombic efficiency of the subsequent cycles is comparable to cells without additives ( Supplementary Fig. 5b ). Prelithiation of graphite flakes by Li x Si–Li 2 O NPs (mass ratio 83:7) shows consistent results, increased first-cycle coulombic efficiency from 87 to 99% ( Supplementary Fig. 6a ). Graphite/LiFePO 4 full cells are used to investigate the effect of Li x Si–Li 2 O particles on full cell performance. The SEM image and half-cell study of LiFePO 4 are shown in Supplementary Fig. 7 . One full cell consists of graphite flake anode prelithiated with Li x Si–Li 2 O particles (graphite flakes:Li x Si–Li 2 O:PVDF=83:7:10), whereas another one consists of an anode with regular graphite flakes (graphite flakes: PVDF=90:10). The cells are measured in the voltage window from 2.5 to 3.8 V at C/10 ( Supplementary Fig. 8a ). The rate and cell capacity are both presented based on the mass of LiFePO 4 in the cathode. The blue voltage profile reveals a plateau between 2.6 and 3.2 V, corresponding to the SEI formation in the anode during charging. After incorporating Li x Si–Li 2 O particles into the anode, the OCV before cycling is about 2.3 V, significantly higher than 0.8 V for regular full cell. As shown by the red voltage profile, the incorporation of Li x Si–Li 2 O NPs compensates the irreversible Li consumption resulting from SEI formation. Accordingly, the first-cycle Coulombic efficiency increases from 77.6 to 90.8%. In the following cycles, the cell with Li x Si–Li 2 O NPs consistently shows a higher capacity than the regular cell ( Supplementary Fig. 8b ). 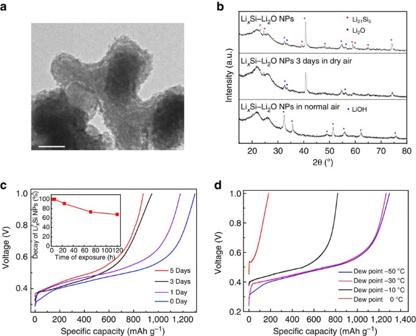Figure 4: Stability of LixSi–Li2O NPs. (a) TEM image of LixSi–Li2O NPs after 3 days of exposure to dry air. Scale bar, 100 nm. (b) XRD patterns of LixSi–Li2O NPs without exposure to dry air, exposed to dry air for 3 days and under ambient conditions. (c) The capacity retention of LixSi–Li2O NPs exposed to dry air with varying durations. The inset shows the trend of capacity decay. (d) The capacity retention of LixSi–Li2O NPs exposed to air at different humidity levels. Stability of Li x Si–Li 2 O NPs Figure 4a is a TEM image to show that the Li x Si–Li 2 O core–shell nanostructure remains after 3 days of exposure to dry air (dew point=−50 °C), although a thicker passivation layer of ~20 nm is observed, as compared with the original 10-nm-thick layer. XRD ( Fig. 4b ) analysis confirms that the sample exposed to dry air for 3 days is still composed of crystalline Li 21 Si 5 and Li 2 O. There is no obvious change in the XRD pattern as compared with the sample without exposure to dry air. The capacities of the Li x Si–Li 2 O NPs exposed to dry air for different numbers of days were studied by delithiating the Li x Si–Li 2 O NPs to 1 V directly ( Fig. 4c ). After exposure to dry air for 1 day, there is 1,175 mAh g −1 capacity, only a 9% decay from time zero. After 5 days of exposure, the Li x Si–Li 2 O NPs still exhibit a capacity of 880 mAh g −1 (red line in Fig. 4c ), showing high capacity retention of 70%. The capacity of the Li x Si–Li 2 O NPs decays slowly with exposure time. The Li x Si–Li 2 O NPs stored in dry air for various durations were added into MCMB graphite to optimize the first-cycle Coulombic efficiency (MCMB:Li x Si–Li 2 O NPs=8:1 by weight). The corresponding cells were tested in the voltage window of 0.005–2 V. The first-cycle voltage profiles of the MCMB/Li x Si–Li 2 O composites ( Supplementary Fig. 9b ) indicate that Li x Si–Li 2 O NPs stored in dry air for 5 days are still active enough to prelithiate MCMB graphite, yielding a 20% improvement in the first-cycle Coulombic efficiency. More attractively, Li x Si–Li 2 O NPs exhibit excellent dry-air stability even at elevated temperatures. MCMB/Li x Si–Li 2 O composites baked at 45°C for 1 h in dry air exhibit a first-cycle Coulombic efficiency of 101.6%. Li x Si–Li 2 O NPs after baking at 65 °C can still effectively prelithiate MCMB graphite to counteract the first-cycle capacity loss as shown in Supplementary Fig. 10 . To test humidity stability, the Li x Si–Li 2 O NPs were stored in an air box with different dew points for 6 h. The capacity of the samples in air with different humidities was studied by discharging the samples to 1 V directly ( Fig. 4d ). The electrochemical performance demonstrates that 6 h of exposure to air with dew point of −30 °C does not affect the capacity. Even in air with a dew point of −10 °C, the Li x Si–Li 2 O NPs still exhibit a capacity of 819 mAh g −1 . However, the Li x Si–Li 2 O NPs were completely converted to LiOH under high humidity, as confirmed by the XRD pattern in Fig. 4b . Figure 4: Stability of Li x Si–Li 2 O NPs. ( a ) TEM image of Li x Si–Li 2 O NPs after 3 days of exposure to dry air. Scale bar, 100 nm. ( b ) XRD patterns of Li x Si–Li 2 O NPs without exposure to dry air, exposed to dry air for 3 days and under ambient conditions. ( c ) The capacity retention of Li x Si–Li 2 O NPs exposed to dry air with varying durations. The inset shows the trend of capacity decay. ( d ) The capacity retention of Li x Si–Li 2 O NPs exposed to air at different humidity levels. Full size image Electrochemical characterization ( Fig. 3b ) shows that the amount of Li preloaded into the Si NPs is 1,310 mAh g −1 for Si. Li is partially consumed to form a Li 2 O passivation layer to protect Li x Si from further oxidation. During the slurry process, DOL decomposes on the surface of the NPs to form a thin layer due to the strong reducing power of Li x Si, further consuming a fraction of the Li. However, the remaining capacity of the Li x Si–Li 2 O NPs is still sufficient as a prelithiation reagent, higher than most Li-rich cathode materials. Compared with the conventional approach of extra loading of cathode materials, prelithiation using Li x Si–Li 2 O NPs more effectively increases the specific energy and energy density of batteries. Li x Si–Li 2 O core–shell NPs can be mixed with various anode materials in the slurry process to achieve high first-cycle Coulombic effieiency. Nanoscale Li x Si particles provide uniform and localized Li distribution to realize fast prelithiation of anode materials. Cycling performance of anode materials is negligibly affected by the addition of prelithiation reagents. The low material loading and particle dimensions are less likely to disturb the structure of the electrode. In addition, void spaces will be formed through delithiaion of the Li x Si additive, which accommodates the volume expansion during the next lithiation process. As shown in Fig. 4c , the capacity retention is 91% after exposure to dry air for 1 day indicating that the Li x Si–Li 2 O NPs are sufficiently stable to go through the battery fabrication process in a dry room. Li x Si–Li 2 O NPs exposed to dry air for 5 days are still active enough to prelithiate MCMB graphite, which yields a 20% improvement in the first-cycle Coulombic efficiency (red curve in Supplementary Fig. 9b ), indicating the potential for long-term storage. We attribute the dry-air stability to the unique core–shell nanostructure. The dense Li 2 O passivation layer has a remarkable effect in preventing Li x Si NPs from thermally oxidizing in dry air. The stabilized Li x Si NPs are still sensitive to moisture. Increasing the stability of the Li x Si alloy in moisture is an important field for future investigations. In summary, we have demonstrated a one-step thermal alloying process to synthesize Li x Si–Li 2 O core–shell NPs without using specialized capital equipment. These NPs exhibit high capacity under dry-air conditions with the protection of the Li 2 O passivation shell, indicating that Li x Si–Li 2 O NPs are potentially compatible with industrial battery fabrication processes in a dry room. Both commercial Si NPs and graphite are prelithiated with Li x Si–Li 2 O NPs, thereby remarkably increasing the first-cycle Coulombic efficiency. It suppresses the undesired consumption of Li from cathode materials during SEI formation. The approach is generally applicable to various anode materials involving complex nanostructures. In addition, the Li x Si alloy also serves as a new anode material with the potential to pair with all high-capacity lithium-free cathodes for next-generation high-energy-density lithium-ion batteries. Synthesis of Li x Si–Li 2 O NPs Si NPs (~50 nm, MTI Inc.) were dried under vacuum for 24 h to remove trapped water. Si NPs (140 mg) were mixed with 154 mg of Li metal foil (99.9%, Alfa Aesar). The Li x Si NPs were synthesized by mixing the Si NPs and lithium foil at 200 °C under mechanical stirring for 6 h in a glove box (Ar-atmosphere, H 2 O level <0.1 p.p.m. and O 2 level <3 p.p.m.). Characterization SEM and TEM images were taken using a FEI XL30 Sirion SEM and a FEI Tecnai G2 F20 X-TWIN, respectively. A FEI Titan 80–300 environmental TEM was employed for EELS mapping collection at an acceleration voltage of 300 kV. The energy resolution of the EELS spectrometer is about 0.9 eV as measured by the full width at half-maximum of the zero-loss peak. EELS mapping data was acquired using a C2 aperture size of 50 mm and a camera length of 48 mm. To minimize sample drift during the STEM EELS mapping, the mapping drift was corrected every 30 pixels. The energy window of the EELS was 40–145 eV for Li (Li K-edge, 54.7 eV) and Si (Si L2, 3 edge 99.2 eV) peaks and 510–615 eV for O (O K-edge, 532 eV) peak. XRD patterns were obtained on a PANalyticalX’Pert, Ni-filtered Cu Kα radiation. Li x Si NPs are sensitive to ambient moisture so the samples were sealed with Kapton tape (DuPont) in the glove box before XRD characterization. Electrochemical measurements Si NPs (~50 nm, MTI Inc.), MCMB graphite (MTI Inc.), carbon black (Super P, TIMCAL, Switzerland) and PVDF binder (Kynar HSV 900) were dried under vacuum for 24 h to remove trapped water. To prepare the working electrodes, various materials were dispersed uniformly in DOL to form a slurry. (Anode materials and mass ratio are based on specific cells.) The slurry was then cast onto a thin copper foil and dried under vacuum. Coin-type cells (2,032) were assembled in an Ar-filled glove box using a Li metal foil as counter/reference electrode. The electrolyte is 1.0 M LiPF 6 in 1:1 w/w ethylene carbonate/DEC (EMD Chemicals), 1 vol % vinylene carbonate and 10 vol% fluoroethylene carbonate (Novolyte Technologies). CV measurements were carried out on a BioLogic VMP3 system. Galvanostatic cycling was carried out using an MTI 8 Channel battery tester. The total mass loading of the Si-based anode was 0.7–1.0 mg cm −2 and a typical total mass loading of the graphite-based anode was 2.0–2.5 mg cm −2 . How to cite this article: Zhao, J. et al . Dry-air-stable lithium silicide–lithium oxide core–shell nanoparticles as high-capacity prelithiation reagents. Nat. Commun. 5:5088 doi: 10.1038/ncomms6088 (2014).